PPM1Dmutations are oncogenic drivers of de novo diffuse midline glioma formation 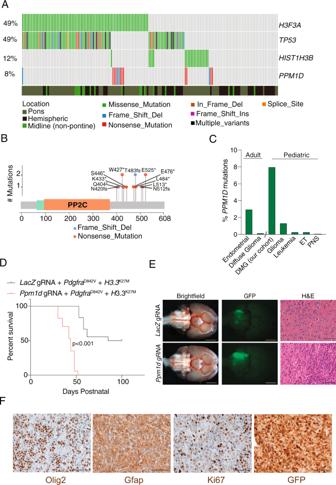Fig. 1:PPM1Dmutations are oncogenic drivers of DMGs. AComutation plot showing alterations in histones (H3F3AandHIST1H3B),TP53,andPPM1Din 170 midline and non-midline gliomas. Variants observed are depicted below.BLollipop plot of recurrent C-terminusPPM1Dtruncating mutations observed in DMGs. The position of nucleotide variants are shown. *Depicts nonsense or truncating alterations.CPercentage of samples withPPM1Dtruncating mutations across different adult and pediatric tumors including DMG dataset from our study.DKaplan–Meier survival curves forH3.3K27M+PdgfraD842VIUE DMG mouse models withLacZgRNA (n= 18) orPpm1dgRNA (n= 17).P< 0.0001 betweenLacZgRNA vsPpm1dgRNA conditions calculated using log-rank Mantel–Cox test.EBrightfield and GFP images ofLacZandPpm1dgRNA IUE DMGs showing GFP-positive tumor regions, and H&E-stained images depicting high-grade glioma histology. Scale bar denotes 2.5 mm (brightfield and GFP) and 50 μm (H&E). Similar staining was performed in a minimum of three independent samples.FPpm1dgRNA IUE DMG sections stained with Olig2, Gfap, Ki67, or GFP. Scale bar denotes 50 μm. Similar staining was performed in a minimum of three independent samples. Source data are provided as a Source Data file. The role of PPM1D mutations in de novo gliomagenesis has not been systematically explored. Here we analyze whole genome sequences of 170 pediatric high-grade gliomas and find that truncating mutations in PPM1D that increase the stability of its phosphatase are clonal driver events in 11% of Diffuse Midline Gliomas (DMGs) and are enriched in primary pontine tumors. Through the development of DMG mouse models, we show that PPM1D mutations potentiate gliomagenesis and that PPM1D phosphatase activity is required for in vivo oncogenesis. Finally, we apply integrative phosphoproteomic and functional genomics assays and find that oncogenic effects of PPM1D truncation converge on regulators of cell cycle, DNA damage response, and p53 pathways, revealing therapeutic vulnerabilities including MDM2 inhibition. Diffuse midline gliomas H3K27-altered (DMG) are universally fatal pediatric brain tumors. In addition to the characteristic histone K27M mutations [1] , [2] , DMGs often harbor alterations in the p53 pathway, including mutations in TP53 itself, as well as PPM1D , a regulator of p53 activity [3] , [4] , [5] , [6] . PPM1D , also known as WIP1, is a PP2C family phosphatase that regulates known members of the DNA damage response (DDR) pathways, most notably p53, as well as other targets such as γ-H2AX, CHK1, ATM, and ATR [7] , [8] , [9] . PPM1D truncating mutations that increase the stability of the phosphatase have also recently been found in clonal hematopoiesis of indeterminate potential (CHIP), where it drives selective outgrowth of the mutant clones in response to cytotoxic chemotherapy [10] , [11] . Previous work in gliomas has largely focused on the role of PPM1D mutation as a driver of radiation resistance and/or evaluated therapeutic vulnerabilities associated with the mutation [12] , [13] , [14] . However, to fully characterize PPM1D as a therapeutic target, a number of questions remain, including its role in DMG oncogenesis, its necessity for the proliferation and maintenance of DMG cells, and finally, its mechanisms of action as an oncogene. In this work, we apply an integrative functional genomic and proteomic approach to systematically examine the role of mutant PPM1D in enhancing DMG oncogenesis and explore its potential as a therapeutic dependency. To this end, we use murine models to demonstrate that endogenous truncation of murine Ppm1d together with histone and Pdgfra mutations is sufficient to drive de novo brainstem glioma formation, as is exogenous expression of truncated human PPM1D ( PPM1D tr). Moreover, we find PPM1D to be necessary for the proliferation of PPM1D -mutant DMGs, and the mechanisms through which PPM1D confers oncogenicity to be primarily mediated through p53, cell cycle, and DDR pathways, creating cellular vulnerabilities that can be therapeutically targeted. Truncating mutations and amplifications of PPM1D are common in histone-mutant midline gliomas and other cancer types PPM1D mutations have previously been reported in gliomas and have been shown to confer resistance to radiation [14] . However, its role as a de novo oncogene to enhance glioma formation has not been explored. To further evaluate the role of PPM1D mutations in gliomagenesis, we first performed a comprehensive analysis of whole-genome sequences (WGS) of 131 pre-treatment pediatric high-grade gliomas (pHGGs). This consisted of 76 DMGs, 58 of which were prototypical diffuse intrinsic pontine gliomas (DIPG) located in the brainstem, and 55 non-midline pHGGs. We also contrasted the whole-genome sequences of these pretreatment tumors to 39 post-treatment pHGGs (34 DMGs including 33 DIPGs and 5 non-midline HGG). Analysis of recurrent single nucleotide variants and copy number alterations confirmed the presence of driver alterations that have been previously described in pHGGs (Supplementary Note 1 ). Consistent with previous reports [3] , [4] , [5] , [6] , we also observed recurrent PPM1D truncating mutations in a subset of pHGG. In our cohort of 170 WGS, we observed PPM1D mutations in 8% of all gliomas (14/170) and 11% of DMG (12/110), with enrichment in DMGs (11/91, Fisher’s exact test, P = 0.056) (Fig. 1A ), and confirmed their anti-correlation with TP53 mutations (Fisher’s exact test, P < 0.0001) (Supplementary Fig. 1A ). All PPM1D mutations were nonsense or frameshift mutations in exons 5 or 6 (Fig. 1B ), resulting in a truncated form of the protein phosphatase WIP1 which has previously been associated with a gain-of-function phenotype [11] , [15] . Fig. 1: PPM1D mutations are oncogenic drivers of DMGs. A Comutation plot showing alterations in histones ( H3F3A and HIST1H3B ), TP53, and PPM1D in 170 midline and non-midline gliomas. Variants observed are depicted below. B Lollipop plot of recurrent C-terminus PPM1D truncating mutations observed in DMGs. The position of nucleotide variants are shown. *Depicts nonsense or truncating alterations. C Percentage of samples with PPM1D truncating mutations across different adult and pediatric tumors including DMG dataset from our study. D Kaplan–Meier survival curves for H3.3 K27M + Pdgfra D842V IUE DMG mouse models with LacZ gRNA ( n = 18) or Ppm1d gRNA ( n = 17). P < 0.0001 between LacZ gRNA vs Ppm1d gRNA conditions calculated using log-rank Mantel–Cox test. E Brightfield and GFP images of LacZ and Ppm1d gRNA IUE DMGs showing GFP-positive tumor regions, and H&E-stained images depicting high-grade glioma histology. Scale bar denotes 2.5 mm (brightfield and GFP) and 50 μm (H&E). Similar staining was performed in a minimum of three independent samples. F Ppm1d gRNA IUE DMG sections stained with Olig2, Gfap, Ki67, or GFP. Scale bar denotes 50 μm. Similar staining was performed in a minimum of three independent samples. Source data are provided as a Source Data file. Full size image The spectrum of cancers associated with PPM1D mutations is distinct in children compared to adults. PPM1D mutations have previously been described in adult myeloid neoplasms including CHIP, myelodysplastic syndrome (MDS), and acute myeloid leukemia (AML) [10] , [11] , but their incidence across other solid cancers is unknown. To assess this, we extended our analysis of PPM1D mutations to include other pediatric and adult cancers (Fig. 1C and Supplementary Note 1 ). Across adult cancers, we observed PPM1D mutations to be recurrent in 3% of endometrial cancers (Fig. 1C and Supplementary Fig. 1B ). In contrast, PPM1D mutations appear to occur predominantly in gliomas in children. Among 41 pediatric cancers encompassing 13 histological subtypes, we found PPM1D truncating mutations in only 0.2% of all tumors, with gliomas being the top tumor type (1.37%) (Fig. 1C ). Within our DMG WGS cohort, we did not observe differences in the frequency of PPM1D mutations between pre- and post-treatment glioma samples (Fisher’s exact test, P = 1), suggesting a role in enhancing de novo glioma formation. Taken together, these data support truncating PPM1D mutations as being contributors of de novo DMG gliomagenesis. Endogenous truncation of Ppm1d exon 6 is sufficient to enhance formation of brainstem gliomas in vivo and confers positive selection in vitro The oncogenic properties of PPM1D mutations have not been previously studied in the primary neural context, particularly in primary neural stem and progenitor cells. To address this, we leveraged In-Utero Electroporation (IUE) to induce C’ terminal truncation of endogenous Ppm1d to evaluate whether this was sufficient to induce glioma formation. We performed brainstem targeted IUE of sgPpm1d exon6 or sgLacZ control to evaluate the effects of PPM1D tr on gliomagenesis. We observed no differences in mice following C’ terminal truncation compared to sgLacZ controls, suggesting that PPM1D tr is insufficient to induce glioma formation as a sole driver alteration (Supplementary Fig. 1C ). However, PPM1D mutations are never observed as sole drivers in DMGs, co-occurring with other alterations including mutated histones and those that result in aberrant growth factor activation. We therefore reasoned that PPM1D mutations may cooperate with other oncogenes to enhance gliomagenesis. To evaluate this, we concurrently electroporated sgPpm1d exon6 with plasmids encoding known drivers of DMGs, including H3.3 K27M and Pdgfra D842V in fetal brainstems of mice. Control IUE (guides targeting LacZ with concurrent H3.3 K27M and Pdgfra D842V PiggyBac plasmids) conditions resulted in a partially penetrant phenotype, with only 50% (9/18) of mice developing neurological symptoms related to tumor, with a median survival of 85 days postnatal (Fig. 1D ). In contrast, C-terminal truncation of Ppm1d by sgPpm1d exon6 was sufficient to generate fully penetrant brainstem gliomas, with all mice developing neurological symptoms (17/17) with a median survival of 44 days, representing a significantly shorter latency ( P < 0.0001 log rank Mantel–Cox test) (Fig. 1D ). Additional sgPpm1d exon6 IUE combinations tested recapitulated prior findings in DNp53 glioma models [16] , where expression of H3.3 K27M and sgPpm1d exon6 was not sufficient to induce gliomas (0/7), while Pdgfra D842V and sgPpm1d exon6 drove efficient tumorigenesis (4/7) with an extended latency (median survival of 83 days postnatal, P < 0.0001 log rank Mantel–Cox test) (Supplementary Fig. 1C ). sgPpm1d exon6 IUE brainstem tumors exhibited features that are also observed in human DMGs. GFP-positive sgPpm1d exon6 IUE brainstem tumors harbored truncations in exon 6 of Ppm1d (Supplementary Fig. 1D–F ) and displayed histopathological traits of high-grade glioma (Fig. 1E, F ). IUE generated murine gliomas showed characteristic histological features seen in human diffuse midline gliomas of the pons (Fig. 1E, F ). Tumors exhibited diffuse single-cell infiltration of the brainstem parenchyma with moderate atypia and mitoses consistent with a high-grade glioma and equivalent to WHO 2016 Grade 3 or 4. Immunohistochemical analysis (Fig. 1F ) showed the expression of GFP was retained in tumor cells uniformly and at high levels and cells retained defining lineage markers of DMG including diffuse Olig2 and Gfap labeling. The proliferation rate by Ki67 staining showed more than 50% of glioma cells positive, similar to human DMGs. We next compared mouse and human DMG transcriptomes. We leveraged RNA-sequencing of sgPpm1d exon6 IUE brainstem tumors to identify highly expressed genes and compared this profile with that of PPM1D -mutant human tumors. 209/14481 genes were found to be highly expressed (Z-score > 2) in the sgPpm1d exon6 tumors (Fig. 2A and Supplementary Data 1 ). 152 of these 209 genes were also highly expressed (Z-score > 2) in PPM1D -mutant human DMGs (Fig. 2B ), representing a significant overlap between the two conditions ( p < 0.0001). Taken together with the histopathological comparisons of these tumors, Ppm1d -mutant IUE brainstem tumors are representative of the tumors observed in human DMG patients. Fig. 2: Expression of human PPM1D tr potentiates DMG formation in vivo and requires the PPM1D phosphatase domain. A Plot showing ranked list of genes based on their expression Z-score in Ppm1d gRNA IUE DMG ( n = 3 tumors). Top genes with expression Z-score > 15 are depicted. B Venn diagram showing highly expressed genes (Z-score > 2) in Ppm1d gRNA IUE DMG ( n = 3), PPM1D -mutant human DMGs ( n = 7), and the overlap between two datasets. Total number of genes analyzed in both datasets is shown outside the box. P < 6.27e−100 calculated using hypergeometric distribution. C Kaplan–Meier survival curves for control ( n = 19), PPM1D tr ( n = 20), and PPM1D tr-D314A ( n = 10) IUE DMG mouse models. P = 0.002 between control vs. PPM1D tr conditions calculated using log-rank Mantel–Cox test. D Brightfield and GFP images of control, PPM1D tr, and PPM1D tr-D314A IUE DMGs showing GFP-positive tumor regions, and H&E-stained images depicting high-grade glioma histology. Scale bar denotes 2.5 mm (brightfield and GFP) and 50 μm (H&E). Similar staining was performed in a minimum of three independent samples. E Control, PPM1D tr, and PPM1D tr-D314A IUE DMG sections stained with Olig2, Gfap, or Ki67. Scale bar denotes 50 μm. F Quantification of the percentage of Ki67-positive cells in Control ( n = 9), PPM1D tr ( n = 8), and PPM1D tr-D314A ( n = 6) IUE DMG models. Data presented as mean ± SEM. P < 0.0001 for both control vs PPM1D tr and PPM1D tr vs PPM1D tr-D314A conditions calculated using two-tailed t -test. Source data are provided as a Source Data file. Full size image C’ terminal truncation of Ppm1d was also sufficient to exert a positive growth advantage in mouse neural stem cells (NSCs) obtained from E14.5 embryos following IUE to induce Ppm1d truncation (Supplementary Fig. 2A, B ) when cultured ex vivo. In the absence of selective pressures, the use of CRISPR-Cas9 is expected to induce out-of-frame indels in a proportion of edits. As these indels would lead to truncation of Ppm1d , we would expect them to confer positive selection pressures. To assess this, we evaluated the change in proportions of truncating Ppm1d events to in-frame INDELS between an early time point (within one month of transfection) and a late time point (following culture for another two months). Indeed, we observed an enrichment of Ppm1d truncating INDELs across time, indicating a positive selection advantage. The cells generated by endogenously truncating Ppm1d at exon 6 ( sgPpm1d ) showed significantly more frameshift modifications compared to cells with non-targeting guides against LacZ ( sgLacZ ) at an early timepoint after establishing the cell line (91.1% ± 0.4% vs 20.9% ± 2.2%, P < 0.05 two-tailed unpaired t -test) (Supplementary Fig. 2C–E ). By the late time point, the proportion of frameshift Ppm1d edits increased to encompass the majority of sequencing reads (99.7% ± 0.2%) in the cells that were transfected by sgPpm1d , but not in the cells transfected with sgLacZ (vs 3.7% ± 3.2%) (Supplementary Fig. 2C–E ), consistent with positive selection of Ppm1d truncating INDELs. Overexpression of PPM1D tr is sufficient to potentiate gliomagenesis and requires the PPM1D phosphatase domain C-terminal PPM1D truncating mutations remove a negative regulatory domain which has been shown to increase the stability of the phosphatase [15] . It is possible that PPM1D mutations are oncogenic specifically through expression of truncated PPM1D , or that simply an increase in wild-type phosphatase activity through over-expression can contribute to oncogenesis. We addressed this question by evaluating whether the exogenous expression of human truncated PPM1D ( PPM1D tr) was also sufficient to promote glioma formation in vivo. Compared to H3.3 K27M and Pdgfra D842V control IUE conditions, the addition of PPM1D tr resulted in enhanced development of fully penetrant gliomas with significantly shortened latency ( P < 0.005, log-rank Mantle-Cox test; median survival 63 vs. 46 days postnatal) (Fig. 2 C and D ). PPM1Dt r IUE DMG models displayed a similar latency to DMG models generated by IUE with the addition of a dominant-negative p53 construct (DN p53 ), which we have previously shown to efficiently cooperate with H3.3 K27M and Pdgfra D842V overexpression [16] (median survival 46 vs. 44 days postnatal, ns, P = 0.37, log-rank Mantle-Cox test) (Supplementary Fig. 3A ). IUE of full-length PPM1D ( PPM1D FL) with H3.3 K27M and Pdgfra D842V plasmids displayed a trend for shortened latency compared to control conditions but did not reach statistical significance (median survival 51 vs. 63 days postnatal, ns, P = 0.14, log-rank Mantle-Cox test) (Supplementary Fig. 3A ). This may reflect known differences in PPM1D FL and PPM1D tr stability [11] , [15] . The PPM1D protein domains that contribute to its oncogenic effects to enhance glioma formation have not been evaluated. To test whether PPM1D phosphatase activity is required for accelerated glioma formation in our models, we performed IUE of H3.3 K27M and Pdgfra D842V plasmids along with a mutant form of PPM1D tr ( PPM1D tr-D314A), that inactivates the phosphatase activity [15] . In contrast to overexpression of PPM1D tr with a wild-type protein phosphatase domain, overexpression of PPM1D tr-D314A was not sufficient to enhance glioma formation relative to IUE of H3.3 K27M and Pdgfra D842V together, and overall survival rates of mice transduced with the phosphatase dead PPM1D tr construct did not differ compared to controls (85 vs 63 days postnatal, ns, P = 0.7, Fig. 2C ). Tumors collected from each IUE condition displayed high-grade glioma histology, expressed Olig2, and contained Gfap-positive reactive astrocytes (Fig. 2E ). Compared to control IUE DMG models, PPM1D tr tumors displayed a significant increase in Ki67-positive proliferating cells (30.59% ± 1.9% vs 12.42% ± 1.5%; P < 0.0001, two-tailed unpaired t-test) (Fig. 2E, F ). Moreover, PPM1D tr-D314A tumors displayed a similar rate of proliferating Ki67-positive cells to that of control IUE conditions (12.6% ± 2.2% vs 12.42% ± 1.5%; ns, P = 0.095 two-tailed unpaired t -test) (Fig. 2E, F ), suggesting that the PPM1D phosphatase activity is required to enhance the growth rate of IUE DMG mouse models. From these experiments, we conclude that the endogenous truncation of the C’ terminal regulatory region of Ppm1d by CRISPR-Cas9 or ectopic expression of truncated PPM1D are similarly sufficient as expression of dominant-negative TP53 to potentiate the in vivo formation of brainstem gliomas in the setting of H3.3 K27M and Pdgfra D842V . Moreover, the PPM1D phosphatase is necessary to enhance DMG formation. Expression of PPM1D is necessary for proliferation of PPM1D -mutant DMG cells Our findings suggest that PPM1D mutations are a clonal driver event that enhances DMG formation. We, therefore, evaluated whether the expression of PPM1D was also necessary for the proliferation of an established PPM1D -mutant DMG cell line BT869 (Supplementary Fig. 4A, B and Supplementary Data 2 ). PPM1D mutant BT869 cells infected with two independent PPM1D -targeting guides exhibited significantly reduced rates of proliferation (mean fold changes from day 0 to day 17, 2.4 ± 0.2 and 1.5 ± 0.1 respectively) compared to those infected with non-targeting control guides (mean fold change 9.1 ± 0.9) ( P < 0.005 for both PPM1D -targeting guides compared to the control guide) (Fig. 3A ). The magnitude of this anti-proliferative effect was similar to our positive control guides which targeted the essential gene EXOSC8 (mean fold change for BT869 from day 0 to day 17, 2.1 ± 0.1, P < 0.005). In contrast, PPM1D -WT DMG lines SU-DIPG-IV and SU-DIPG-XIII were not dependent on PPM1D expression (SU-DIPG-IV: mean fold changes from day 0 to day 22 for sgRNA PPM1D #1 and #2 and sgRNA LacZ 77.5 ± 3.3, 82.8 ± 5.4, and 76.3 ± 18.6 respectively, P = 0.9 and P = 0.6 respectively. SU-DIPG-XIII: mean fold changes from day 0 to day 11 for sgRNA PPM1D #1 and #2 and sgRNA LacZ 17.6 ± 1.4, 16.4 ± 3.9, and 20.6 ± 1.5 respectively, P = 0.2 and P = 0.4 respectively) (Fig. 3B and Supplementary Fig. 4C ). Fig. 3: PPM1D is a dependency in PPM1D tr but not PPM1D -WT cell lines. A Fold change in proliferation compared to day 0 of PPM1D -mutant patient-derived cell line (PDCL) BT869 after transfection with PPM1D -KO sgRNAs, nontargeting ( LacZ ) sgRNA, or lethal ( EXOSC8 ) sgRNA. Growth curves show mean ± SEM from three replicates and are representative of three independent experiments. P = 0.0021, 0.0011, and 0.0016 for PPM1D -KO #1, PPM1D -KO #2, and EXOSC8 respectively calculated using two-tailed t -test. B Growth of PPM1D -WT PDCL SU-DIPG-IV after transfection with indicated sgRNAs. Growth curves show mean ± SEM from three replicates and are representative of three independent experiments. P = 0.8963, 0.5524, and 0.0335 for PPM1D -KO #1, PPM1D -KO #2, and EXOSC8 respectively calculated using two-tailed t -test. C Probability of PPM1D dependency as determined by pooled CRISPR-cas9 assays across 558 cancer cell lines, subgrouped according to their TP53 mutation and PPM1D copy-number status. Bounds of the box represent the IQR, center represents the median, and the bounds of the whiskers represent 1.5 times IQR. P < 0.0001 for TP53 WT/ PPM1D non-amplified cells vs both TP53 -mutant/ PPM1D -amplified and TP53 -mutant/ PPM1D non-amplified cells and P < 0.01 for TP53 WT/ PPM1D non-amplified cells vs TP53 WT/ PPM1D -amplified cells using Kruskal–Wallis test. D Growth of PPM1D -mutant colon cell line HCT116 after transfection with indicated sgRNAs. Growth curves show mean ± SEM from three replicates and are representative of three independent experiments. P = 0.0015, 0.0010, and 0.0059 for PPM1D -KO #1, PPM1D -KO #2, and EXOSC8 respectively calculated using two-tailed t -test. E – F Growth of PPM1D -mutant DMG cell lines BT869 ( E ) and SF7761 ( F ) after treatment with vehicle control (NT), 10 μM of GSK2830371 (PPM1Di), 2 Gy of ionizing radiation treatment (RT), or the combination of both (GSK + RT). Growth curves show mean ± SEM from at least three replicates and are representative of three independent experiments. BT869: P = 4.90083E-06, 2.18655E−07, 3.83657E−11, 2.8877E−11, and 1.1625E−06 for NT vs PPM1Di, NT vs RT, NT vs PPM1Di + RT, RT vs PPM1Di + RT, and PPM1Di vs PPM1D + RT respectively calculated using two-tailed t -test; SF7761: P = 0.003367278, 1.17616E−05, 5.59401E−08, 1.5694E−08, and 2.698E−05 for NT vs PPM1Di, NT vs RT, NT vs PPM1Di + RT, RT vs PPM1Di + RT, and PPM1Di vs PPM1D + RT respectively calculated using two-tailed t -test. Source data are provided as a Source Data file. Full size image To further complement our findings, we used a next-generation sequencing (NGS)-based competition assay to track the selection of PPM1D -disrupted alleles relative to unedited or in-frame modifications. In this assay, the relative abundance of loss-of-function CRISPR-Cas9 mediated edits can be used to determine whether the expression of PPM1D is necessary for proliferation. In the PPM1D -mutant line BT869, the proportion of loss-of-function PPM1D alterations decreased over time (33% ± 2.2% at early time point vs. 16% ± 2.4% at late time point) (Supplementary Fig. 4D ), suggesting that PPM1D -mutant DMG cells require the expression of PPM1D for proliferation. However, we did not observe a similar decrease in loss-of-function alterations of PPM1D in PPM1D -WT cell lines SU-DIPG-IV and SU-DIPG-XIII (Supplementary Fig. 4E, F ). Our finding that PPM1D is necessary for PPM1D -mutant DMGs extended to other PPM1D -expressing cancers. We examined whether PPM1D dependency was linked to genetic activation of PPM1D using pooled CRISPR-cas9 assays across 558 cancer cell lines [17] , [18] . We hypothesized that TP53 -WT cell lines would be more dependent on PPM1D than TP53 -mutant cell lines because of PPM1D’s role in opposing p53 function. As expected, lines with wild-type TP53 were significantly more dependent on PPM1D than TP53 -mutant lines ( P < 0.0001) (Fig. 3C ). Among TP53 -WT lines, PPM1D copy-number gain was associated with significantly higher probability of dependency on PPM1D ( P < 0.01) (Fig. 3C ). We conclude that PPM1D is required for the proliferation of p53 wild-type cell lines, particularly those that harbor PPM1D activating genetic alterations. However, the cell lines in this dataset did not fully represent PPM1D -mutant DMGs as almost all non-DMG cell lines containing PPM1D tr mutations also harbored TP53 mutations (7/8 lines) which may be acquired during cell passaging [19] . We therefore also validated this dependency in a PPM1D tr colon cancer cell line (HCT116), which does not harbor a TP53 mutation. Similar to our observations in PPM1D -mutant DMGs, disruption of PPM1D using guides directed to the PPM1D tr phosphatase domain resulted in reduced growth compared to controls (mean fold changes from day 0 to day 6 for PPM1D sgRNA #1, PPM1D sgRNA #2, sgRNA LacZ , and sgRNA EXOSC8 were 11.4 ± 0.5, 10.3 ± 0.4, 23 ± 1.4, 6.4 ± 2.8 respectively, P < 0.005 for both PPM1D guides and P < 0.05 for sg EXOSC8 ) (Fig. 3D ). Taken together, these findings confirm PPM1D expression to be necessary for the proliferation of PPM1D -mutant cancer cells, nominating it as a potential therapeutic target across multiple lineages. We also found small-molecule inhibition of PPM1D to further suppress the viability of PPM1D -mutant DMG cells in the presence of ionizing radiation (IR). GSK2830371 is a tool PPM1D inhibitor that has been shown to antagonize PPM1D function in cancer cell lines [20] , [21] . We treated PPM1D -mutant DMG cell lines BT869 and SF7661 with 10 μM of GSK2830371 (GSK), 2 Gy of IR, or the combination of both. Inhibition of PPM1D with GSK or treatment with  IR by themselves decreased the viability of the cells compared to no treatment (NT) control (BT869: mean fold change from day 0 to 5: 4.6 ± 0.2 for NT, 6.5 ± 0.1 for GSK ( P < 0.0001), and 8.6 ± 0.1 ( P < 0.0001) for IR respectively (Fig. 3E ); SF7761 mean fold change from day 0 to 5: 2.4 ± 0.1 for NT, 2.2 ± 0.0 for GSK ( P < 0.0005), and 2.7 ± 0.0 for IR ( P < 0.0001) respectively (Fig. 3F ). However, the combination of these two treatments further decreased the viability of these cells over time (BT869: mean fold change at day 5 1.4 ± 0.1 ( P < 0.0001); SF7761 mean fold change at day 5 1.5 ± 0.0 ( P < 0.0001)) (Fig. 3E, F ), exhibiting a possible additive effect. These findings suggest that the induction of DNA-damage through IR further accentuates the necessity of PPM1D expression in PPM1D -mutant DMGs. PPM1D tr suppresses apoptosis and potentiates progression of cells through the G1/S checkpoint following ionizing radiation treatment PPM1D has been shown to have multiple substrates that regulate cellular functions, including regulation of cell cycle progression, DDR, and the induction of apoptosis [8] , [9] , [10] , [11] . We, therefore, reasoned that PPM1D tr may act through these pathways to enhance the cellular proliferation of PPM1D -mutant DMGs. To evaluate the effects of PPM1D tr overexpression, we transduced in vitro primary mouse neural stem cell models (mNSCs) that ectopically express K27M mutant H3F3A ( H3 K27M) with PPM1D tr-, PPM1D FL-, or a green fluorescent protein (GFP) control-expressing vector. We were able to achieve successful consistent overexpression of PPM1D tr but not PPM1D FL (Supplementary Fig. 5A ), likely because full-length PPM1D is actively degraded as previously reported [11] , [15] . Expression of PPM1D tr was associated with attenuated apoptosis and more rapid cell cycling after IR treatment. We treated our mNSC models with IR and assessed the percentage of apoptotic and cycling cells using flow-cytometry analysis of Annexin V/Propidium Iodide (PI) and BrdU/7-AAD respectively (Supplementary Fig. 5B–G ). Compared to GFP controls, PPM1D tr overexpression led to significantly lower rates of apoptosis at baseline (11.5% ± 1.3% and 6.1% ± 0.9% respectively; P < 0.05), and with even greater effects 24 h after 8 Gy of IR treatment (22.9% ± 2.3% and 13.3% ± 2.4%, respectively; P < 0.05) (Fig. 4A ). PPM1D FL overexpression did not lead to a significant decrease in apoptosis at baseline, but decreased apoptosis 24 h after 8 Gy of IR treatment (12.8 ± 2.3; P < 0.05). At 24 h post-IR treatment, the majority of GFP expressing cells remained in G0/G1 (77.9% ± 7.1%), while only 6.3% ± 1.5% had re-entered cell-cycling and were in S-phase. However, cells expressing PPM1D FL and PPM1D tr exhibited a more rapid progression through the G1/S checkpoint, with 18% ± 1.4 and 17% ± 1.5% of cells respectively, observed to be in S phase ( P < 0.05 and P < 0.005 respectively) (Fig. 4B ). The suppression of apoptosis and G1/S cell cycle checkpoint by PPM1D FL suggests that even low levels of PPM1D overexpression might be enough to confer this difference in the context of DNA damage. Fig. 4: PPM1D suppresses apoptosis, DDR, and p53 pathways. Apoptosis and cell cycle responses were assessed in isogenic mouse neural stem cells (mNSCs) overexpressing H3F3A K27M ( H3 K27M) mutation plus either eGFP (vector control), full-length PPM1D ( PPM1D FL), or C-terminus truncated PPM1D ( PPM1D tr) ( A – B ). A Cells were treated with 8 Gy of ionizing radiation (RT) or no treatment (NT) for 24 h, incubated with Annexin V-APC and Propidium Iodide (PI), and analyzed using flow cytometry. The total percentage of Annexin V positive cells representing both early and late apoptotic cells are shown. Data presented as mean ± SEM from three biological replicates. P = 0.027, 0.318, 0.044, 0.037 for GFP vs PPM1D tr (NT), GFP vs PPM1D FL (NT), GFP vs PPM1D tr (RT) and GFP vs PPM1D -FL (RT) conditions respectively calculated using two-tailed t-test. B Cells were treated with 8 Gy RT for 24 h and integration of BrdU was assessed to determine the percentage of cells in S-phase. Anti-BrdU APC and 7-AAD DNA staining were used to distinguish cells in each stage of the cell cycle. Data presented as mean ± SEM from three biological replicates. P = 0.276, 0.090 0.008, 0.005, 0.543, 0.848 for GFP vs PPM1D FL (G0/G1) GFP vs PPM1D tr (G0/1), GFP vs PPM1D FL (S) GFP vs PPM1D tr (S), GFP vs PPM1D FL (G2/M) GFP vs PPM1D tr (G2/M) conditions respectively calculated using two-tailed t -test. C Cells were treated with 8 Gy of RT and lysates were collected at baseline (NT), 1 and 5 h post-RT respectively, and probed with the indicated antibodies. Three independent experiments were performed with similar results. D PPM1D -mutant patient-derived DMG cell lines BT869 and SF7761 were treated with 10 μM of GSK2830371 (PPM1Di) and/or 8 Gy of RT for 1 and 5 h, lysed and probed with indicated antibodies. Three independent experiments were performed with similar results. E Volcano plot showing differentially expressed genes in BT869 and SF7761 DMG cells ( n = 3 per cell line per condition) treated with 10 μM of GSK2830371 (PPM1Di) for 5 h compared to vehicle treatment. Genes in the p53 signaling pathway are labeled. F GSEA enrichment plots of two p53 related pathways significantly enriched (FDR < 0.25) after inhibition of PPM1D in BT869 and SF7761 cells. Source data are provided as a Source Data file. Full size image PPM1D truncations have been shown to stabilize PPM1D, leading to enhanced dephosphorylation of its substrates [11] , [15] . Moreover, we observed the PPM1D phosphatase to be necessary for PPM1D tr to enhance DMG formation. We, therefore, reasoned that PPM1D truncations associated with PPM1D -mutant gliomas may also exhibit the enhanced activity of the PPM1D phosphatase, targeting known substrates in the DDR and cell cycle pathways. Expression of PPM1D tr was associated with reduced phosphorylation of PPM1D substrates in the DDR pathway, in both primary mNSC models and patient-derived DMG cell lines. We treated mNSCs generated by endogenously truncating Ppm1d at exon 6 ( sgPpm1d ) or non-targeting guides against LacZ ( sgLacZ ) with IR and assessed response to DNA damage using previously described markers γ-H2AX and p-p53 (Ser15) at both baseline and five-hours post-IR treatment (Supplementary Fig. 6A ). We observed decreased phosphorylation of these markers in mNSCs with truncated Ppm1d in both conditions ( P < 0.05) (Supplementary Fig. 6A, B ). We also found similar decrease in phosphorylation of these markers in mNSCs overexpressing PPM1D tr compared to those overexpressing GFP ( P < 0.05) (Fig. 4C and Supplementary Fig. 6C ). Next, we leveraged the tool PPM1D inhibitor to evaluate whether suppression of PPM1D was sufficient to reverse this phenotype. We treated two patient-derived PPM1D -mutant DMG cell lines, BT869 and SF7761 with the PPM1D inhibitor GSK2830371 at 10 μM. Treatment with GSK2830371 by itself for 5 h increased the levels of γ-H2AX and p-p53 (Ser15) in PPM1D -mutant DMG lines ( P < 0.05) and this effect was further enhanced by IR treatment (Fig. 4D and Supplementary Fig. 6D ). Taken together, these data indicate that PPM1D tr confers changes on cellular processes that converge on regulation of cell-cycle progression and DDR including induction of apoptosis. PPM1D tr inhibition leads to increased transcription of TP53 and DDR pathways in PPM1D mutant DMGs To evaluate the transcriptional changes conferred by PPM1Dtr in DMGs, we treated PPM1D -mutant DMGs BT869 and SF7761 with 10 μM of GSK2830371 and compared their gene-expression profiles to those of DMSO treated cells at 1, 5, and 24 h post treatment. We observed 114, 368, and 219 genes to be differentially expressed at 1, 5, and 24 h post treatment (LFC > 2, FDR < 0.25) in the GSK2830371 treated cells compared to vehicle controls (Fig. 4E , Supplementary Fig. 7A and Supplementary Data 3 ). The most significantly upregulated genes five hours post treatment included the chemokine CXCL8 , ZBTB32 , a member of the ZBTB family of transcription factors and TRIML2 , which has been reported to enhance p53 SUMOylation [22] , while the most downregulated genes included the monocarboxylate transporter SLC16A3 and MYOD1 , a bHLH transcription factor most well-known for its role in regulating myogenic differentiation [23] (Supplementary Data 3 ). At a pathway level, 353/1836, 176/1453, and 90/1858 pathways were significantly upregulated (FDR < 0.25) in the GSK2830371 treated condition relative to DMSO condition at 1, 5, and 24h time points respectively. Five hours post treatment, 8 of the 10 most significantly upregulated pathways included gene-sets associated with TP53 -signaling and one with DDR. Moreover, of the remaining 166 pathways, another 10 were also related to TP53 signaling, 12 with cell cycle regulation, and 9 with DDR (Fig. 4F , Supplementary Fig. 7B, C and Supplementary Data 4 ). Ten of these signaling pathways remained upregulated at the 24 h time point. PPM1Dtr dephosphorylates substrates in the DDR and cell cycle regulation pathways in PPM1D -mutant DMGs To further evaluate the magnitude of the effects of PPM1Dtr on proteins involved in the DNA damage and cell cycle responses relative to the entire phosphoproteome, we leveraged multiplexed quantitative mass-spectrometry approaches to systematically identify all substrates that are differentially altered in the presence of PPM1Dtr. We first quantitatively identified proteins and phosphosites associated with the PPM1D phosphatase function in the PPM1D -mutant cell line BT869. Cells treated with 10 μM of the PPM1D inhibitor GSK2830371 for 5 h exhibited differential alteration of 184 phosphosites relative to DMSO controls (LFC > 1 and FDR < 0.01) (Fig. 5A and Supplementary Data 5 ). Some of these phosphosites included CHEK2 (S303, S478), TP53 (S15, S9 S15), TP53B1 (S1073, S1764), MDC1 (S955), SMC3 (S1067, S1065 S1067), MCM3 (S726, S580), and RAD18 (S142, S403) (Fig. 5A and Supplementary Data 5 ). Functional protein association of the top 50 differentially altered proteins using STRING [24] revealed that these targets were enriched for 89 biological processes (FDR < 0.05), including DNA repair, cell cycle, DNA damage checkpoint, DNA damage response by p53, G1/S transition of the mitotic cell cycle, and G2/M transition of the mitotic cell cycle (Fig. 5B, C and Supplementary Data 6 ). Fig. 5: Phosphoproteomic analysis of PPM1D substrates in PPM1D -mutant cell lines. A Patient-derived PPM1D -mutant DMG cell line BT869 was treated with 10 μM of the PPM1D inhibitor GSK2830371 (or DMSO vehicle control) for 5 hours to suppress the PPM1D phosphatase following which phosphoproteomic profiling was performed. A Heatmap of top 50 differentially altered phosphosites (LFC > 1 and FDR < 0.01) between GSK2830371 treated (PPM1Di) and vehicle-treated (DMSO) samples is shown. Experiments were performed in triplicates. B Pathway enrichment analysis using STRING reveals significantly associated biological pathways among phosphosites shown in ( A ) and, ( C ) Associated core interactome following PPM1D suppression. D Significantly enriched or downregulated pathways (FDR < 0.05) revealed by PTM-SEA analysis of the phosphosites between the two conditions. Positive and negative enrichment scores correspond to biological pathways upregulated and downregulated respectively in GSK2830371 treated (PPM1Di) samples compared to vehicle-treated (DMSO) samples. E Motif analysis showing conserved amino acids flanking 97 confidently localized phosphorylation sites that are upregulated upon PPM1D inhibition in BT869 cells (LFC > 1, FDR < 0.01) and their associated probability of occurrence at that position. Full size image However, these analyses are based on the identity of the protein and do not consider the status of specific phosphorylation sites, which confer functional significance. To address this, we also performed enrichment analysis of post-translational modification (PTM) sites using the recently developed PTM-SEA method [25] . We found 17 PTM pathways to be significantly altered (FDR < 0.05), including seven pathways related to cell cycle and CDK signaling (CDK1, CDK2, CK2A2/CSNK2A2, CK2A1/CSNK2A1, AurA/AURKA, and AurB/AURKB, TTK), four pathways related to DDR such as ATM, ATR, and CHEK2 signaling, and another two pathways associated with receptor tyrosine kinase signaling (Fig. 5D ). We next applied a recently published method CausalPath [26] to integrate our phosphoproteomic data with literature knowledge to generate causal hypotheses from the data. This analysis also indicated several DNA repair genes (ATM, ATR, MDC1, MRE11) to be activated upon PPM1D inhibition (Supplementary Fig. 8A ). Some of the observed phosphorylations of TP53 and TRIM28 are identified to be a consequence of PPM1D inhibition (Supplementary Fig. 8A ). We also observed some inhibitory sites on PPM1D (S54 and S85) to be downregulated, possibly due to some negative feedback on PPM1D (Supplementary Fig. 8A ). Furthermore, sequence motif analysis identified a conserved SQ motif among putative PPM1D-dependent phosphorylation events ( P = 1.6e−49) (Fig. 5E ), further supporting the role of PPM1D in response to DNA damage [27] . Consistent with the previous reports [11] , we also observed an overrepresentation of glutamic acid at position +2 ( P = 4.2e−19). We also characterized the phosphoproteome of mNSCs transduced to express PPM1Dtr. We identified 1420 unique phosphosites to be differentially altered in PPM1Dtr cells compared to GFP cells (LFC > 1 and FDR < 0.01), including phosphosites in Tp53bp1 (S571, S1750), Mdm2 (T286 S288, S183), Smc3 (S1067, S1065 S1067), and Atrx (S822) (Supplementary Fig. 8B and Supplementary Data 7 ). We also found 18 PTM pathways to be significantly altered in PPM1Dtr cells compared to GFP (FDR < 0.25), including three pathways related to CDK signaling (CDK2, CDK4, and CDK5), consistent with our observations in the phosphoproteome of human DMG (Supplementary Fig. 8C ). Taken together, these findings confirm that expression of PPM1Dtr is predominantly associated with altered phosphorylation in the regulators of TP53-related pathways, including cell cycle and DDR pathways. Cell cycle, TP53 associated, and DDR pathways represent genetic dependencies in PPM1D tr-expressing mNSCs Our findings nominate PPM1D tr as being sufficient for enhancement of glioma formation and necessary for proliferation of PPM1D tr cells. Moreover, we find DDR, TP53, and cell cycle pathways to be associated with the functional effects of PPM1D tr. We, therefore, reasoned that these pathways would also be necessary for the proliferation of PPM1D tr-expressing cells. To evaluate this, we performed a genome-scale CRISPR/Cas9 loss-of-function screen in mNSCs overexpressing PPM1D tr to identify genes whose ablation resulted in a decreased fitness of the cells. We found the ablation of 19 genes to result in a positive selection advantage (LFC > 1, FDR < 0.25), while ablation of another 1588 genes suppressed their growth (LFC < −2, FDR < 0.25) (Fig. 6A , Supplementary Data 8 ). However, 893 of these latter genes have been identified as pan-essential dependencies across all cell types, leaving 695 genes that are more likely to be PPM1D tr-associated dependencies. Gene-set enrichment analysis (GSEA) of the genes identified as not being pan-essential revealed 241 canonical pathway gene sets (FDR < 0.25) to be significantly enriched among this set. At least 38 of these gene sets included pathways representing cell cycle/cell cycle checkpoints, DDR, and the TP53 pathway (Fig. 6B , Supplementary Data 9 ). We observed similar findings when the analyses were repeated with more stringent thresholds (Supplementary Data 9 ). In contrast, no gene-sets (0/19 significant gene sets, FDR < 0.25) in these pathways were enriched in dependencies identified in wild-type NSCs (Supplementary Data 10 ). Fig. 6: MDM2 inhibition is a dependency in PPM1D -mutant DMGs. A Volcano plot of genetic dependencies associated with mNSC overexpressing PPM1D tr as revealed by genome-wide loss of function CRISPR-cas9 screen. Average LFC of normalized reads for each gene across three replicate experiments, and associated p-values are shown. A negative LFC represents depletion of guides across the assay. Genes that reach the FDR cutoff of 0.25 are labeled in red. B Gene-sets significantly enriched (FDR < 0.05) within the dependencies associated with PPM1D tr-expressing mNSCs following removal of pan-essential genes. C Genes ranked by Pearson correlation of PPM1D dependency (CERES score) against dependency of all other genes (CERES score) across 738 cancer cell lines. D Correlation between PPM1D dependency (CERES score) and response to Nutlin-3 treatment (AUC) across 309 cancer cell lines. Pearson correlation coefficient and associated two-tailed p-value of the coefficient are shown. Error bars represent 95% confidence interval. E RT-qPCR quantification of MDM2 expression in BT869 cell line infected with shRNA targeting GFP or MDM2 (two independent shRNA). Results show mean ± SEM for four replicates and are representative of three independent experiments. P = 6.66e−13 and 3.34e−11 for GFP vs shRNA MDM2 #1 and GFP vs shRNA MDM2 #2 respectively using two-tailed t -test. F Growth of BT869 cells with MDM2 knockdown from ( E ). Growth curves are mean ± SEM for at least three replicates and are representative of three independent experiments. P = 3.67e−08 and 6.34e−10 for GFP vs shRNA MDM2 #1 and GFP vs shRNA MDM2 #2 at 156 h respectively using two-tailed t -test. G – I Drug response curves for a panel of two PPM1D -mutant and two PPM1D -WT DMG cell lines treated with different concentrations of MDM2 inhibitors AMG232 ( G ), RG7388 ( H ), and Nutlin-3 ( I ) as indicated. Data presented as mean ± SEM from three independent experiments. Source data are provided as a Source Data file. Full size image These results support the expression of cell cycle, DDR, and TP53 pathway members as being necessary for the proliferation of PPM1D tr-expressing mNSCs. However, cancer cells frequently harbor other genetic alterations that can also influence vulnerabilities associated with oncogenes that are not in our primary mNSC models. We, therefore, sought to expand our analyses to include cancer cell lines, leveraging genome-scale CRISPR-Cas9 screens completed across 558 independent models [17] . We calculated pairwise Pearson correlations between PPM1D dependency and dependency on all other genes within the DepMap dataset (Fig. 6C ) and found cell cycle checkpoint and TP53 -associated DNA repair genes to be most strongly associated with PPM1D dependency. Negative regulators of TP53 signaling and PPM1D substrates MDM2 and MDM4 were the top dependencies that correlated with PPM1D dependency (Fig. 6C and Supplementary Fig. 9A ). PPM1D expression also correlated with MDM2 dependency across all cell lines (Supplementary Fig. 9B ). However, cell cycle checkpoints CHEK1 , CHEK2 , ATM , and ATR were anti-correlated with PPM1D dependency. In contrast, dependency on Atm and Chek2 were associated with PPM1D tr expression in our mNSC models. Unlike cancer cell lines, mNSCs have intact TP53 and cell cycle checkpoints. We speculate that other interventions that induce DNA damage may be required to unmask these dependencies in cancer cells that harbor other alterations beyond PPM1D mutations. We validated MDM2 to be a genetic dependency in PPM1D -mutant BT869 DMG cells. Suppression of MDM2 expression by two different short hairpin RNA (shRNA) led to significantly reduced rates of proliferation (mean fold changes from hours 30 to hours 192 were 18.2 ± 0.4 and 13.4 ± 0.3 respectively) compared to those infected with non-targeting control shRNA against GFP (mean fold change 29 ± 0.6) ( P < 0.0001 for both MDM2 -targeting shRNA compared to the GFP shRNA) (Fig. 6E, F ). Consistent with the genetic data, PPM1D -dependent cancer cells also tended to be sensitive to pharmacologic inhibition of MDM2 using the MDM2 inhibitor Nutlin-3 (Pearson 0.38, P < 10 −21 ) (Fig. 6D ). This finding extended to PPM1D -mutant DMG cells. We evaluated the efficacy of the older generation MDM2 inhibitor Nutlin-3 and two newer generation MDM2 inhibitors, AMG232 and RG7388 [28] , [29] , across a panel of four patient-derived PPM1D -mutant and PPM1D -WT DMG cell lines. PPM1D -mutant lines (BT869 and SF7761) were more sensitive to all three drugs compared to the PPM1D -WT cells (SU-DIPG-XIII and SU-DIPG-XVII) ( P < 0.0005 and P < 0.05 for AMG232 and RG7388 respectively) (Fig. 6G–I and Supplementary Data 11 ). We obtained a similar result in an analysis of AMG232 and RG7388 treatment across another independent cohort of five patient-derived DMG lines, including three PPM1D -mutant lines (HSJD-DIPG-007, HSJD-DIPG-008, and HSJD-DIPG-014A) and two PPM1D -WT TP53 mutant cell lines (QCTB-R059 and ICR-B184) ( P < 0.05 and P = 0.05 for AMG232 and RG7388 respectively) (Supplementary Fig. 9C–D and Supplementary Data 11 ). We also evaluated the sensitivity of our endogenous Ppm1d truncated mouse NSC lines. Within these isogenic cell lines, Ppm1d truncated cells tended to be more sensitive to AMG232 treatment compared to WT ( sgLacZ ) control cells (Supplementary Fig. 9E ). Taken together, these results support the hypothesis that MDM2 inhibition is an actionable therapeutic vulnerability in PPM1D -mutant DMGs. Our integrative analyses with an array of models and genomic, proteomic, and functional assays (Fig. 7 ), including the development of mouse models of PPM1D -mutant DMGs, nominate PPM1D as an oncogenic driver in de novo DMG. We confirm previous reports suggesting truncating mutations in exon 6 of PPM1D are clonal driver events in DMG [30] , [31] and show that they are sufficient to enhance de novo glioma formation. Moreover, we find expression of PPM1D tr to be necessary for proliferation of PPM1D -mutant DMG cells, and, applying orthogonal approaches, we find that these effects are largely mediated through PPM1D tr’s role in regulating TP53 , DDR and cell cycle pathways. Fig. 7: Integrative analysis of PPM1D -mutant DMG models. Schematic depicting the overall method and findings of the study. Top panel: an array of models used in the study including biopsy of DMG tumors, de novo mouse models of PPM1D driven DMG using in utero electroporation, and in vitro models including patient-derived cell lines. Middle panel: integrative approach employing whole-genome sequencing of patient tumors, gene expression analysis, proteomics, and phosphoproteomics screens, and CRISPR screens used to study the function and mechanism of PPM1D mutation in DMG. Bottom panel: convergence of the oncogenic function of PPM1Dtr on p53, cell cycle and DDR pathways using the integrative approach in the middle panel. Full size image Using in utero electroporation to examine the role of mutant PPM1D in vivo, our data provide direct evidence that PPM1D truncations actively participate in de novo DMG development. 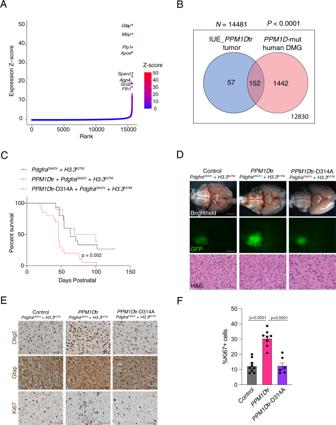Fig. 2: Expression of humanPPM1Dtr potentiates DMG formation in vivo and requires thePPM1Dphosphatase domain. APlot showing ranked list of genes based on their expression Z-score inPpm1dgRNA IUE DMG (n= 3 tumors). Top genes with expression Z-score > 15 are depicted.BVenn diagram showing highly expressed genes (Z-score > 2) inPpm1dgRNA IUE DMG (n= 3),PPM1D-mutant human DMGs (n= 7), and the overlap between two datasets. Total number of genes analyzed in both datasets is shown outside the box.P< 6.27e−100 calculated using hypergeometric distribution.CKaplan–Meier survival curves for control (n= 19),PPM1Dtr (n= 20), andPPM1Dtr-D314A (n= 10) IUE DMG mouse models.P= 0.002 between control vs.PPM1Dtr conditions calculated using log-rank Mantel–Cox test.DBrightfield and GFP images of control,PPM1Dtr, andPPM1Dtr-D314A IUE DMGs showing GFP-positive tumor regions, and H&E-stained images depicting high-grade glioma histology. Scale bar denotes 2.5 mm (brightfield and GFP) and 50 μm (H&E). Similar staining was performed in a minimum of three independent samples.EControl,PPM1Dtr, andPPM1Dtr-D314A IUE DMG sections stained with Olig2, Gfap, or Ki67. Scale bar denotes 50 μm.FQuantification of the percentage of Ki67-positive cells in Control (n= 9),PPM1Dtr (n= 8), andPPM1Dtr-D314A (n= 6) IUE DMG models. Data presented as mean ± SEM.P< 0.0001 for both control vsPPM1Dtr andPPM1Dtr vsPPM1Dtr-D314A conditions calculated using two-tailedt-test. Source data are provided as a Source Data file. Previous studies have leveraged flank implants of immortalized human astrocytes with endogenous PPM1D truncations, or orthotopic implants of murine glioma cells exogenously expressing PPM1D tr [13] , [14] but have not assessed the direct contribution of mutant PPM1D to the transformation of neural stem/progenitor cells into DMG. We demonstrate that when paired with expression of Pdgfra and histone K27M mutations, either truncation of endogenous Ppm1d or exogenous expression of PPM1Dtr is sufficient to enhance gliomagenesis to a similar degree as p53 loss of function, and that the PPM1D phosphatase is necessary for this phenotype. While expression of Pdgfra , histone K27M or Ppm1d mutations alone do not result in high-grade glioma formation, the combination of Pdgfra and histone K27M mutations together results in a partially penetrant phenotype. This is likely due to the ability of histone K27M mutations to decrease/suppress Cdkn2a (p16) expression [16] , [32] . The presence of PPM1D or TP53 mutations in histone K27M mutant DMGs suggests additional alterations in the cell cycle and DDR are necessary for DMG progression, and likely cooperate with decreased p16 expression. We have generated mouse models of genetically engineered, PPM1D -driven DMG, including one that faithfully recapitulates endogenous PPM1D truncation as observed in human gliomas. One of the major limitations in developing new therapeutic approaches that target candidate genetic drivers is the availability of disease-relevant model systems. IUE DMG mouse models provide an in vivo platform to assess and optimize therapeutic approaches, including challenges associated with drug penetration across the blood-brain barrier [33] , [34] and resistance to radiotherapy, which is the only therapy that provides temporary relief for DMG patients [35] . With the development of Ppm1d mutant DMG mouse models, which represent to our knowledge the only DMG/DIPG mouse models that do not include Trp53 or Cdkn2a loss of function [32] , [36] , a direct assessment of p53 function in therapeutic response can be performed. Our data in PPM1D -mutant patient-derived DMG cultures nominates therapeutic targets (i.e. MDM2) that reactivate TP53 . In addition, interactions of glioma cells with the tumor microenvironment can be fully evaluated since IUE mouse models develop as de novo tumors in immune-competent mice. In this study, multiple assays indicated that PPM1D tr cooperatively drives DMG primarily by opposing the key functions of p53. First, genetic analyses found that PPM1D tr mutations are mutually exclusive with TP53 mutations in DMG suggesting that these mutations have overlapping oncogenic functions. Second, in vivo and in vitro tumor initiation studies found PPM1D tr to be sufficient to replace dominant-negative TP53 to enhance glioma formation in vivo and abrogate TP53 -mediated G1/M cell cycle arrest and apoptosis in vitro. Third, genetic and phosphoproteomic assays of DMG model systems identified TP53 , cell cycle and cell cycle checkpoints, and DDR pathways—all of which are also functions of p53—as the primary pathways affected by perturbations of PPM1D tr. Similarly, prior studies found genetic exclusivity between PPM1D and TP53 alterations [5] , [6] and identified PPM1D tr-associated chemotherapy/radiation resistance and clonal expansion in glial and hematopoietic compartments [10] , [11] . However, several clues point to possible additional functions of PPM1D truncation in glioma development. For instance, PPM1D tr but not TP53 mutation co-occurs with PIK3CA mutations in DMG, suggesting a possible interaction with the MAPK and mTOR pathways and its potential role in tumorigenesis. Future studies will seek to fully dissect these possible mechanistic interactions. The current results nominate PPM1D as a therapeutic target for DMGs, both in solo PPM1D -targeting therapy and by enhancing DDR activators such as γ-H2AX and p-p53 (Ser15) when combined with DNA-damaging agents including radiation and chemotherapy. These findings are consistent with previous reports that PPM1D is a dependency when suppressed by shRNA or tool PPM1D inhibitors [12] , [14] . While there are currently no clinically relevant PPM1D inhibitors, tool compounds that inhibit its phosphatase domain have been developed, providing optimism for future efforts to generate compounds with favorable pharmacokinetic and brain penetrant properties [37] , [38] . Notably, TP53 -mutant/ PPM1D -WT DMGs would not be predicted to benefit from PPM1D inhibition since PPM1D acts upstream of p53. These findings imply that PPM1D and TP53 mutation status should be considered as biomarkers for response in investigations of PPM1D -directed therapies in DMG. Our data also identify nodes in the PPM1D genetic network as therapeutically actionable dependencies in PPM1D tr DMGs. While our study implies that PPM1D tr and TP53 loss of function have overlapping oncogenic functions, tumors with either alteration are likely to harbor different genetic dependencies. For instance, the protein-ubiquitin ligase MDM2 which targets p53 for degradation is well-known to be a dependency in TP53 wild-type cancers, but inhibition of MDM2 is ineffective in cancers that already harbor loss of p53 function [28] , [29] , [39] . Importantly, emerging data suggest that p53 wild-type cancers that are driven by PPM1D gain of function are still susceptible to MDM2 inhibition [40] . Consistent with this observation, our current studies identify MDM2 dependency as a potentially actionable feature of PPM1D-truncated DMGs, leading to genotyping for PPM1D as an inclusion criterion for a clinical trial of an MDM2 inhibitor in pediatric cancers (NCT03654716). However, multiple additional therapeutic avenues remain largely unexplored. For example, future studies should investigate additional nodes of the PPM1D molecular genetic network that could be therapeutically targeted both individually and in combination in PPM1D tr DMG. Ethics statement The WGS and RNA-seq data of pHGGs were obtained from Dubois et al. (unpublished) study. New data were generated from tumors collected with informed consent under the Dana-Farber Cancer Institute Tissue Banking Protocol (DFCI 10417) or from tumors collected for research studies on the DIPG BATs clinical trial (NCT01182350). Ethics approval was granted by the relevant human IRB of Dana-Farber Cancer Institute (DFCI) and collaborating institutions. All patients provided informed consent prior to collection of samples or were analyzed as de-identified samples with specific IRB waiver of informed consent. Cell line authentication and mycoplasma testing SU-DIPG-IV, SU-DIPG-XIII, SU-DIPG-XVII were obtained from Dr. Michelle Monje at Stanford University, and BT869 cell lines were obtained from the DFCI Center for Patient-Derived Models (CPDM). HCT116 and HEK293T were obtained from Broad Institute’s Cancer Cell Line Factory (CCLF). SF7761 cell line was purchased from Sigma Aldrich (SCC126). HSJD-DIPG-007, HSJD-DIPG-008, HSJD-DIPG-014A, ICR-B184, and QCTB-R059 cells were obtained from Drs. Chris Jones and Angel Carcaboso. mNSCs used for overexpression studies were obtained from Dr. Charles Stiles at DFCI and were generated as previously described [41] , [42] , Cells were routinely fingerprinted or sequenced for identity validation and tested (at least every 3 months) for mycoplasma infection using the MycoAlert Mycoplasma Detection Kit (Lonza, LT07-318), according to the manufacturer’s instructions. Whole-genome sequencing and processing We analyzed recently generated WGS from pediatric high-grade gliomas (pHGG), including DMG, and their matched normal [43] . Additional WGS data analyzed were downloaded from previously published studies [3] , [4] , [44] , [45] . This dataset consisted of 131 pre-treatment pHGGs (76 DMGs and 55 non-midline pHGGs) and 39 post-treatment pHGGs (34 DMGs and 5 non-midline pHGGs). Among patients with available demographic information, there were equal proportions of males and females and the age ranged from 0.1 years to 31 years with mean age of 9.49 years. For whole-genome sequencing, genomic DNA extracted from the samples were fragmented and libraries were prepared. Alignment of reads to the human reference genome GRCh37 (hg19) was performed using the Burrows-Wheeler Aligner (BWA) [46] ; duplicates were marked using SAMtools and Picard. Recalibration of base quality score to control for biases was performed using the Genome Analysis Toolkit (GATK) [47] . Mutation and copy number analysis Single nucleotide variants (SNVs) and short indels were called using GATK4-MuTect2 pipeline and visual inspections were performed in the Integrative Genomics Viewer (IGV) [48] . MutSig2CV was applied to detect significantly recurrent mutations [49] . Copy number alterations were evaluated using the GATK4 somatic CNV pipeline. Copy number calls were purity and ploidy normalized using ABSOLUTE [50] . GISTIC 2.0 was used to identify recurrent copy-number alterations [51] , [52] . All analyses were performed within Broad Institute’s Firecloud platform. Maftools R package was used to generate mutation plots used in the figure [53] . TCGA analysis Analysis of PPM1D and its associated alterations across several cancer types in the TCGA dataset was performed using the cBioPortal [54] , [55] , TumorPortal [49] , and Tumorscape [56] software. The data from these portals were accessed on August 2019 for adult tumors and January 2021 for pediatric tumors. Vector constructions H3F3A K27M, PPM1D full-length ( PPM1D FL), PPM1D truncated ( PPM1D tr, AA 1–426), PPM1D truncated phosphatase-dead ( PPM1D tr-D314A) constructs were synthesized as Gateway-compatible entry clones with GenScript. These gene sequences in the Gateway entry vectors were then cloned into the pLX313 ( H3F3A K27M) and pLX311 ( PPM1D FL, PPM1D tr, and PPM1D tr-D314A) destination vectors using Gateway LR Clonase II reaction (Life Technologies, 11791-020). pLX311- GFP and pLX313- GFP vectors were purchased from the Broad Genetics Perturbation Platform (GPP). For the PPM1D constructs, V5 was N-terminally tagged in the entry clone. For the remaining vectors, V5 in the destination vector was cloned to be in frame with the construct. In utero electroporation DMG mouse models All mouse work was done according to institutional and IACUC review boards (University of Cincinnati). Time pregnant (e13–14) CD1-ICR mice (Charles Rivers) were used for all experiments. Mice were socially housed in PIV cages on a 14/10-h dark/light cycle. Temperatures were maintained between 68–75 ˚F, with 45–65% relative humidity. In utero electroporation was performed as previously described [16] . Briefly, ~1 μL of concentrated DNA mixtures (1 μg/μL per plasmid) containing 0.05% Fast Green (Sigma) was injected into the fourth ventricle of embryos using a pulled glass capillary pipette. Injected embryos were electroporated by applying 5 square pulses (45 V, 50 ms pulses with 950 ms intervals; BTX ECM830) with the positive electrode of a 3 mm tweezer electrodes directed towards the lower rhombic lip of the fourth ventricle. Embryos were returned to the abdominal cavity, incision sutured, and the female monitored until fully recovered. Electroporated pups were identified by bioluminescent imaging (IVIS Xenogen) and monitored for neurological symptoms related to tumor burden. For histopathology, 10% formalin-fixed brains were transferred to 70% ethanol before paraffin embedding. 5 μm thick sections were prepared on a microtome (Lecia) and processed for haematoxlin-eosin (H&E) staining. Immunohistochemistry for noted antigens were performed at the CCHMC pathology core using the automated Ventana Symphony and BenchMark stainers. Antibodies include Olig2 (Millipore, Ab9610) (1:2000), Gfap (Cell Signaling, 12389) (1:1000), GFP (Thermo Fisher, A11122) (1:1000), and Ki67 (Cell Signaling, 9129) (1:2000) at indicated dilutions. PiggyBac transposon donor plasmids encoding V5-tagged PPM1D tr, PPM1D tr-D314A, and PPM1D FL were generated by InFusion cloning into EcoRI digested PB-CAG-Ires-Luciferase (Takara, USA). H3F3A K27M, Pdgfra D842V, and DNp53 PiggyBac donor plasmids were described previously [16] . sgRNA sequences were designed using CHOPCHOP [57] and cloned into the all-in-one CRISPR-Cas9 plasmid pX458 (Addgene, 48138) using previously described protocols [58] . 20nt-NGG gRNA-PAM sequences include: Ppm1d gRNA#1: CGTCGGTGCTTCTTCATAAG-GGG, Ppm1d gRNA#2: TTCGACTTAAGCCATTTCGT-CGG, and LacZ gRNA: TGCGAATACGCCCACGCGAT-CGG. Cutting efficiency of Ppm1d exon6 DNA was validated using the guide-it sgRNA screening system according to the manufactures instructions (Takara, USA). The following primers were used to PCR amplify fragments of Ppm1d exon 6 targeted by gRNAs: Fwd- TCCAGACTGTAGTGATGACCTCA, Rvs- TCAACATTAGCCCTGCTGTCACA. For TIDE analysis, Ppm1d exon6 sequence was amplified using the aforementioned primers using gDNA template from cells or tumor samples electroporated with Ppm1d gRNA#1 or LacZ gRNA. PCRs were submitted to the CCHMC DNA sequencing and genotyping core for sanger sequencing. Trace files were analyzed by TIDE [59] to determine the quantitative spectrum of indels around the Ppm1d cut site. For next-generation sequencing, the sequence surrounding the Ppm1d exon6 cut site was PCR amplified using the following primers: Fwd- GCTCAAGAAGTTGAAAGAACCC, Rvs-CATCTCAGCACACACACACT. PCR products were submitted to the DFCI MBCF for NGS sequencing and the results were analyzed using the CRISPResso2 tool [60] . Amplicon sequencing for CRISPR editing characterization DNA was extracted using DNA Mini Kit (Qiagen, 51306) and the target region in mouse Ppm1d was amplified by PCR (EMD Millipore) using the following primers: Ppm1d -F GCTCAAGAAGTTGAAAGAACCC; Ppm1d -R CATCTCAGCACACACACACT. The successful amplification of this region was validated by running the purified PCR product in 1.5% agarose gel. After validation, amplicons were submitted for NGS sequencing to the DFCI MBCF. The sequencing FastQ files were analyzed and the percent of modified reads (both in-frame and frameshift) were calculated using the CRISPREsso2 software [60] . Bulk RNA sequencing RNA extraction was performed using the RNAeasy kit (Qiagen, 74104). Once the samples passed initial QC analysis for quantity and quality, library prep was performed using Roche Kapa mRNA Hyper Prep and sequenced using the Illumina NovaSeq 6000 platform at DFCI MBCF. The sequencing FastQ files were aligned and counted using STAR [61] . The raw count matrix was normalized and Z-scored in IUE mouse tumors and human DMG for comparison. For PPM1D -mutant cell lines BT869 and SF7761, differential expression parameters were calculated using the DESeq2 pipeline [62] . Data from both cell lines were averaged for this analysis and genes with a total combined count of <10 were ignored. The normalized counts produced by DESeq2 were also used for pathway enrichment analysis using GSEA [63] . Calculation of significance of overlap of highly expressed genes between the human and mouse DMGs was calculated using the web tool available at http://nemates.org/MA/progs/overlap_stats.html . Culturing of mNSCs mNSCs were maintained in ultra-low attachment flasks in culture medium with 1:1 ratio of DMEM/F-12 (Invitrogen, 11330-032) and Neurobasal A (Invitrogen, 10888-022) consisting of 1% each of HEPES Buffer Solution 1 M, sodium pyruvate solution 100 nM, non-essential amino acids solution 10 mM, Glutamax-I Supplement and Penicillin/Streptomycin solution. The media was supplemented with B27 Minus Vitamin A (Invitrogen, 12587-010), epidermal growth factor (EGF; StemCell Tech. Inc., 78006), fibroblast growth factor (FGF; GF003, StemCell Tech. Inc., 78003) and heparin solution, 0.2% (StemCell Tech. Inc., 07980). Cells were dissociated using Accutase (StemCell Tech. Inc., 07922) and passaged every 3 or 4 days. Stable expression of H3F3AK27M, PPM1D FL, and PPM1D tr in mNSCs HEK293T cells were transfected with 10 μg of lentiviral expression vectors with packaging plasmids encoding PSPAX2 and VSVG using Lipofectamine 3000 (L3000075). Lentivirus-containing supernatant was collected 24 h after transfection, pooled, and concentrated using the Lenti X-Concentrator (Takara, 631231) according to the manufacturer’s instructions. Target mNSCs were infected using a spin protocol (931 g for 120 min at 30 °C with no polybrene). Cells were selected using Blasticidin selection in pLX311 vector expressing cells (1 μg/mL) and hygromycin selection (200 μg/mL; Life Technologies, 7246) in pLX313 vector expressing cells 24 h after the infection. Culturing of patient-derived DMG and other cell lines All DMG cell lines used in the study (except for SF7761) were cultured in ultra-low attachment flasks in culture medium with 1:1 ratio of DMEM/F-12 (Invitrogen, 11330-032) and Neurobasal A (Invitrogen, 10888-022) and ten percent each of HEPES Buffer Solution 1 M (Thermo Fisher, 15630080), Sodium Pyruvate solution 100 nM (Life Technologies, 11360070), MEM non-essential amino acids solution 10 mM (Thermo Fisher, 11140050), Glutamax-I Supplement (Thermo Fisher, 35050061), and Penicillin/Streptomycin solution (Life Technologies, 15140122). The media was supplemented with B27 Minus Vitamin A (Invitrogen, 12587-010), epidermal growth factor (EGF; StemCell Tech. Inc., 78006), fibroblast growth factor (FGF; GF003, StemCell Tech., Inc., 78003) and heparin solution, 0.2% (StemCell Tech. Inc., 07980), as well as PDGF-AA (Shenandoah Biotech, 100-16) and PDGF-BB (Shenandoah Biotech, 100-18). SF7761 cell line was cultured in medium with Neurobasal A (Invitrogen, 10888-022) and N-2 Supplement (Invitrogen, 17502), further supplemented with B27 Minus Vitamin A (Invitrogen, 12587-010), epidermal growth factor (EGF; StemCell Tech. Inc., 78006), fibroblast growth factor (FGF; GF003, StemCell Tech. Inc., 78003) and heparin solution, 0.2% (StemCell Tech. Inc., 07980). Cells were dissociated using Accutase (StemCell Tech. Inc., 07922) and passaged every 3 or 4 days. MDM2 knockdown BT869 cells were infected with lentiviral plasmids expressing shRNA against human MDM2 or GFP as a control. The following shRNA sequences were used: MDM2 #1, CTCTCGACTCAGAAGATTATA; MDM2 #2, ATCAACTTCTAGTAGCATTAT; GFP, GCAAGCTGACCCTGAAGTTCAT. One day after infection, cells were started selection in 1 μg/mL puromycin. Two days post selection, cells were plated into 96-well plates and the proliferation rates were analyzed over time using spheroid assay in the Incucyte live cell imaging system. Knockdown of MDM2 was validated using qRT-PCR. Quantitative reverse transcription PCR RNA was extracted using the RNeasy Mini kit (Qiagen) and subjected to on-column DNase treatment. cDNA was synthesized with the Superscript II Reverse Transcriptase kit (Life Technologies) with no–reverse-transcriptase samples serving as negative controls. Gene expression was quantified by Power Sybr Green Master Mix (Applied Biosystems). MDM2 expression values were normalized to Beta-Actin and the fold change was calculated by the DDCt method by comparing to the parental cells and scaling to the average of the vector control condition. Primers used in our studies are as follows: h-MDM2 -F: GCAGTGAATCTACAGGGACGC; h-MDM2 -R: ATCCTGATCCAACCAATCACC; Beta-Actin-F: ACGTGGACATCCGCAAAGAC; Beta-Actin-R: CAA GAAAGGGTGTAACGCAACTA PPM1D knockout experiments SU-DIPG-IV, SU-DIPG-XIII, HCT116, and BT869 cells were infected with plasmids expressing cas9 and two independent guides against PPM1D exon 6, LacZ , or known an essential gene EXOSC8 . The following gRNA sequences were used: lacZ , TGCGAATACGCCCACGCGAT; PPM1D #1 GCCAGTGTGGTCATCATTCG, PPM1D #2, GAACGAATCGAAGGACTTGG; EXOSC8 CGGAATCTCGATGAACACAG. Cell lines were first transfected with LentiBlastCas9 [64] and selected with Blasticidin (Thermo Fisher, A1113903) to generate stable pools of cells expressing Cas9. Cells were then transfected with LentiGuidePuro plasmids [64] as described above to express the indicated gRNAs. After two days, cells were introduced to 400 ng/μL puromycin selection. For growth assays, cells were seeded into 96-well plates in triplicate on day 4 after transfection. CellTiterGlo assays were performed on Day 0 and on at least 3 additional time points based on the growth dynamics of the cell line being assayed. For serial monitoring of PPM1D gene disruption by NGS, transfected cells were added to T75 flasks and serially passaged. gDNA was isolated and subjected to PCR to amplify a 150–300 bp region encompassing the guide site of interest. To confirm EXOSC8 cutting, the following primers were used: AGCTGCAGAGTGTTTCTTTCA and AGAGCAAAGTAAATGAAAAGCCCAA. To confirm PPM1D #1 cutting, the following primers were used: GCGGAATGGCCAAAGACTAT and CACCAAGTCCTTCGATTCGT. For PPM1D #2, the following primers were used: CAACTGCCAGTGTGGTCATC and AAGGGACAGTAGTAGGTCAATTTCA. NGS was performed at the MGH CCIB to assess for the percentage of copies of PPM1D that were uncut, those that had PPM1D damaging edits, and those that had in-frame edits. Protein extraction and immunoblotting Cells were lysed in RIPA (radioimmunoprecipitation) buffer containing protease and phosphatase inhibitors on ice and sonicated for 10 one-second pulses. Lysate was centrifuged at 13,000 × g for 15 min and the supernatant was harvested. Supernatant was quantified with the Pierce 660 nm Protein Assay (Thermo Fisher, 22660) and mixed with 4X LDS Sample loading buffer (Invitrogen, NP0008) and heated at 70 °C for 10 min. Equal amounts of samples were loaded and separated by SDS-PAGE on 4–12% Bis-Tris gradient gels. Antibodies against the following proteins were used with indicated dilutions: Phospho-p53 (Ser15) (D4S1H) Rabbit mAb (Rodent Specific) (Cell Signaling, 12571) (1:200), p53 (1C12) Mouse mAB (Cell Signaling, 2524) (1:200), Phospho-Histone (H2A.X) (Ser139) (20E3) Rabbit mAB (1:1000), Rabbit Monoclonal Histone H2A.X Antibody (Cell Signaling, 2595) (1:1000), p53 Antibody (DO-1) mouse monoclonal (Santa Cruz Biotechnologies, sc126) (1:200), Monoclonal Anti-Vinculin antibody produced in mouse (Sigma, V9131) (1:1000), Anti-V5 Antibody (Thermo Fisher, R960-25) (1:1000), Phopho-p53 (Ser15) Antibody (Cell Signaling, 9284) (1:500). After transferring, the blots were blocked in Odyssey Blocking Buffer (Li-Cor, 927-40125) for one hour at room temperature. Blots were put in primary antibody at 4 °C overnight, and secondary antibody for 2 h at room temperature. Anti-mouse IgG, HRP-linked antibody (Cell Signaling, 7076) (1:10,000) and Anti-rabbit IgG, HRP-linked antibody (Cell Signaling, 7074) (1:10,000) were used as secondary antibodies against mouse and rabbit primary antibodies respectively. The blots were washed in 1X TBST three times for 15 min total between each step. To develop the blots, they were saturated in SuperSignal West Pico PLUS Chemiluminescent Substrate (Thermo Fisher, 34578). Visualization was performed using the Fujifilm LAS-3000 Imaging System. Flow cytometry for apoptosis and cell cycle mNSCs were treated with 8 Gy of ionizing radiation and the experiments were performed 24 h post treatment. Annexin V-APC (Thermo Fisher, A35110) and Propidium iodide (Thermo Fisher, NC9699940) were used to determine the proportion of early and late apoptotic cells as previously described [65] . The proportion of cells in different phases of the cell cycle was determined by flow cytometric assessment using the APC BRDU/7-AAD Flow Kit (BD biosciences, 556454) as per the manufacturer’s instructions. GSK2830371 and ionizing radiation treatment of DMG cell lines PPM1D -mutant DMG cell lines BT869 and SF776 were treated with vehicle control (DMSO), 10 μM of PPM1D inhibitor GSK2830371 (MedChemExpress, 5140), 2 Gy ionizing radiation treatment, or the combination of both. Cells were seeded at a density of 1000 cells per well in 96-well ULA plates. Each biological replicate had six technical replicates for each cell line. The proliferation rates were analyzed over time using spheroid assay in the Incucyte live cell imaging system. An unpaired t-test assuming equal variance was conducted to compare the fold change values between different conditions at day 5 of the experiment. Sample processing for phosphoproteomic analysis mNSC overexpressing GFP, PPM1D full-length or PPM1D tr were grown in ultra-low attachment chambers (Corning) in three technical replicates per condition. Similarly, patient-derived DMG cell line BT869 was treated with either DMSO or 10 μM of PPM1D inhibitor GSK2830371 in triplicates for 5 h. Both mNSC and BT869 cell pellets were prepared for MS analysis using an optimized workflow [66] employing a tandem mass tag (TMT) isobaric labeling strategy. Briefly, all cell pellets were lysed in an 8 M urea lysis buffer, followed by reduction, alkylation, and digestion using LysC followed by trypsin overnight. Samples were desalted using reverse phase C18 SepPak cartridges (Waters Corp.) and 400 μg aliquots were prepared for isobaric labeling. The TMT 10-plex included mNSC samples (three replicates for each experimental condition) along with a pooled reference sample that consisted of all the mNSC samples. The experiment using BT869 samples was a TMT 6-plex and contained three replicates for each experimental condition. Labeling was done following a reduced TMT protocol [67] . After confirming 98% or greater label incorporation, reactions were quenched; samples for each plex were mixed together, desalted, then fractionated and concatenated into 24 fractions. Five percent of each fraction was taken for global proteome analysis by liquid chromatography-mass spectrometry (LC-MS/MS). 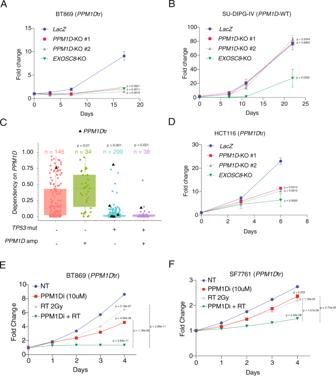Fig. 3:PPM1Dis a dependency inPPM1Dtr but notPPM1D-WT cell lines. AFold change in proliferation compared to day 0 ofPPM1D-mutant patient-derived cell line (PDCL) BT869 after transfection withPPM1D-KO sgRNAs, nontargeting (LacZ) sgRNA, or lethal (EXOSC8) sgRNA. Growth curves show mean ± SEM from three replicates and are representative of three independent experiments.P= 0.0021, 0.0011, and 0.0016 forPPM1D-KO #1,PPM1D-KO #2, andEXOSC8respectively calculated using two-tailedt-test.BGrowth ofPPM1D-WT PDCL SU-DIPG-IV after transfection with indicated sgRNAs. Growth curves show mean ± SEM from three replicates and are representative of three independent experiments.P= 0.8963, 0.5524, and 0.0335 forPPM1D-KO #1,PPM1D-KO #2, andEXOSC8respectively calculated using two-tailedt-test.CProbability ofPPM1Ddependency as determined by pooled CRISPR-cas9 assays across 558 cancer cell lines, subgrouped according to theirTP53mutation andPPM1Dcopy-number status. Bounds of the box represent the IQR, center represents the median, and the bounds of the whiskers represent 1.5 times IQR.P< 0.0001 forTP53WT/PPM1Dnon-amplified cells vs bothTP53-mutant/PPM1D-amplified andTP53-mutant/PPM1Dnon-amplified cells andP< 0.01 forTP53WT/PPM1Dnon-amplified cells vsTP53WT/PPM1D-amplified cells using Kruskal–Wallis test.DGrowth ofPPM1D-mutant colon cell line HCT116 after transfection with indicated sgRNAs. Growth curves show mean ± SEM from three replicates and are representative of three independent experiments.P= 0.0015, 0.0010, and 0.0059 forPPM1D-KO #1,PPM1D-KO #2, andEXOSC8respectively calculated using two-tailedt-test.E–FGrowth ofPPM1D-mutant DMG cell lines BT869 (E) and SF7761 (F) after treatment with vehicle control (NT), 10 μM of GSK2830371 (PPM1Di), 2 Gy of ionizing radiation treatment (RT), or the combination of both (GSK + RT). Growth curves show mean ± SEM from at least three replicates and are representative of three independent experiments. BT869:P= 4.90083E-06, 2.18655E−07, 3.83657E−11, 2.8877E−11, and 1.1625E−06 for NT vs PPM1Di, NT vs RT, NT vs PPM1Di + RT, RT vs PPM1Di + RT, and PPM1Di vs PPM1D + RT respectively calculated using two-tailedt-test; SF7761:P= 0.003367278, 1.17616E−05, 5.59401E−08, 1.5694E−08, and 2.698E−05 for NT vs PPM1Di, NT vs RT, NT vs PPM1Di + RT, RT vs PPM1Di + RT, and PPM1Di vs PPM1D + RT respectively calculated using two-tailedt-test. Source data are provided as a Source Data file. The remaining 95% of the 24 fractions was then concatenated down to 12 fractions that were enriched for phosphopeptides by immobilized metal (Fe3+) affinity chromatography (IMAC) [66] . Mass spectrometry and data analysis The proteome and phosphoproteome fractions were analyzed as described previously [66] on either a Q Exactive Plus mass spectrometer (proteome) or a Q Exactive HF-X mass spectrometer (phosphoproteome) coupled with an Easy-nLC 1200 LC system (Thermo Fisher Scientific). Data were searched on the Spectrum Mill MS Proteomics Workbench (Broad Institute) using either a mouse or human database that contained 47069 and 69062 entrees downloaded from Uniprot.org on 12/28/2017 and 08/05/2020, respectively. The Spectrum Mill generated proteome level export from the proteome dataset filtered for proteins identified by two or more peptides and the phosphosite level export from the phosphoproteome dataset were used for further statistical analyses. Protein and phosphosite quantification were achieved by taking the ratio of TMT reporter ions for each sample over the TMT reporter ion for the pooled reference channel for the TMT10 mouse experiment or the median of all channels for the TMT6 human samples. TMT10 and TMT6 reporter ion intensities were corrected for isotopic impurities in the Spectrum Mill protein/peptide summary module using the afRICA correction method which implements determinant calculations according to Cramer’s Rule [68] and correction factors obtained from the reagent manufacturer’s certificate of analysis ( https://www.thermofisher.com/order/catalog/product/90406 ) for lot numbers TE270709 and UC280588 respectively. After performing median-MAD normalization, a moderated two-sample t-test was applied to both the mouse and human datasets to compare GFP and PPM1D tr (mouse), or drug and DMSO (human) samples. Benjamini-Hochberg corrected p -value thresholds were used to assess significantly regulated proteins and phosphosites between experimental conditions. Enrichment of biological pathways among the proteins with top 50 significantly altered phosphosites (LFC < 1, FDR < 0.05) in the human data was performed using STRING [24] . PTM signature enrichment analysis Enrichment analysis of phosphoproteome datasets was performed by Post Translational Modification-Signature Enrichment Analysis (PTM-SEA) [25] using results of moderated two-sample t -test. A table was generated for both mouse and human datasets that included all identified phosphosites with an assigned value that incorporated the FDR corrected p -value along with the direction of fold change. These phosphosite tables were searched against curated site-centric databases in PTMsigDB, version 1.9.0 which included 130 and 558 unique signatures for mouse and human, respectively. CausalPath analysis CausalPath [26] is an analysis tool for proteomic datasets that generates causal hypotheses by aligning the observed changes with literature knowledge. We applied CausalPath with 0.05 FDR threshold on phosphoproteomic differential abundances and generated 51 result relations. We inserted inhibition of PPM1D as a custom hypothesis and used 0.05 FDR threshold for network significance calculations. Sequence motif analysis Sequence motif logos depicting the conservation of amino acid residues around confidently localized phosphorylation sites (Spectrum Mill VML score > 1.1) were generated with the “motifStack” Bioconductor R-package. Putative PPM1D-dependent phosphorylation sites were defined by stringent criteria to mitigate the impact of potential secondary, non-PPM1D-dependent phosphorylation events (log FC > 1, adjusted p < 0.01) resulting in 97 upregulated phosphorylation sites upon PPM1D inhibition. Background frequencies of amino acids were calculated from the human proteome database (UniProt, downloaded 05 Aug 2020). The significance of the conserved occurrence of amino acids in a sequence window of ±7 amino acids around phosphorylation sites was calculated by the Fisher exact test using the sequence windows of all detected and localized phosphorylation sites as background ( N = 23 740). Cas9 activity assay in mNSC overexpressing PPM1D tr Cas9 activity was assessed in mNSC overexpressing PPM1D tr in preparation for the genome-wide loss of function screen. 2 × 10 6 cells were seeded in one well of a 12-well plate, then spin-infected with pLX311-GFP virus. Cells were flow-sorted for GFP-positive cells and then spin-infected with an all-in-one vector of sgGFP and Cas9. Cells were selected for 48 h with puromycin (commencing 48 h post-infection). Cas9 activity was confirmed with flow analyzer, measuring percent decrease in GFP positive cell fraction as previously described [17] . Determination of infection conditions for CRISPR pooled screens Optimal infection conditions were determined in order to achieve 30–50% infection efficiency, corresponding to a multiplicity of infection (MOI) of ~0.5–1, by infecting cells with different virus volumes. No-spin infections were performed in ultra-low attachment T25 flasks (Corning) with 6 × 10 5 cells/mL in conditioned media per flask. Each virus volume was seeded in duplicate flasks, and cells were then incubated at 37 °C. After 6 h, an additional 3 mL of ‘2X’ media per flask was added to dilute the virus. Approximately 30 h after infection, one flask per virus volume was supplemented with 3 mL of ‘2X’ media per flask; the other flask per virus volume was supplemented with 3 mL of ‘2X’ media per flask and with a final concentration of 0.5 μg/mL puromycin. Cells were counted 3 days post selection to determine the infection efficiency, comparing survival with and without puromycin selection. Volumes of virus that yielded ~30–50% infection efficiency were used for screening. CRISPR pooled proliferation screens The lentiviral barcoded ‘Brie’ library used in the primary screen contains 79,633 sgRNAs, which includes an average of 4 guides per gene and 1000 non-targeting control guides. The ‘Brie’ library was cloned into the pXPR_BRD023 vector, which contains Cas9 under an EFS promotor. Genome-scale infections were performed in three replicates with the predetermined volume of virus in the same no-spin format as the viral titrations described above in ultra-low attachment 1-layer chambers (Corning). Infections were performed with enough cells per replicate in order to achieve a representation of at least 500 cells per sgRNA per replicate following puromycin selection (~4 × 10 7 surviving cells per replicate). Approximately 6 h after infection, ‘2X’ media was added to each chamber, and 30 h after infection, cells were selected with puromycin for three days to remove uninfected cells. After the selection was complete, ~4 × 10 7 cells per replicate were passaged to maintain representation of the library. Cells were passaged every 3–4 days and harvested ~25 days after infection. Genomic DNA (gDNA) was isolated using Maxi kits according to the manufacturer’s protocol (Machery-Nagel). PCR and sequencing were performed as previously described [69] , [70] . Samples were sequenced on a HiSeq2000 (Illumina). For analysis, the read counts were normalized to reads per million and then log 2 transformed. The log 2 fold-change of each sgRNA was determined relative to the plasmid DNA of the library for each biological replicate. The log 2 fold-change, p -value, and FDR adjusted p -value across the three biological replicates were calculated using the Broad Institute’s Hypergeometric analysis. For the pathway enrichment analysis among the significantly enriched or depleted genes, GSEA pre-ranked [63] , [71] was used with all the gene sets in the c2.cp curated list in the MSigDB collections. MDM2 inhibition experiments MDM2i assays in the patient-derived cell lines (BT869, SF7761, SU-DIPG-XIII, and SU-DIPG-XVII) were performed by seeding 1000 cells per well in a 96-well white bottomed plate (Corning 3917) with DMSO controls. The MDM2i assays were performed using Nutlin-3 (Catalog No. HY-50696), Idasanutlin (RG7388 Catalog No. HY-15676), AMG232 (Catalog No. HY-12296). The drugs were plated in 1:3 serial dilutions, with 10 concentrations ranging from 0 μM to 50 μM with three biological replicates. Each biological replicate had three technical replicates for each cell line. Total number of viable cells were determined by trypan blue assays. After three days of incubation (72 h), luminescence measurements of ATP content using CellTiterGlo (Promega) were performed as a marker of cell viability. The measurements were normalized to the DMSO control with 0 μM drug. Patient-derived cultures HSJD-DIPG-007 ( H3F3A K27M, PPM1D P428fs), HSJD-DIPG-008 ( H3F3A K27M, PPM1D 1286delG), HSJD-DIPG-014A ( H3F3A K27M, PPM1D 1451dupT, ICR-B184 ( HIST1H3C K27M, PPM1D wild-type), QCTB-R059 ( H3F3A K27M, PPM1D wild-type) were grown as neurospheres in stem cell media consisting of Dulbecco’s Modified Eagles Medium: Nutrient Mixture F12 (DMEM/F12), Neurobasal-A Medium, HEPES Buffer Solution 1 M, sodium pyruvate solution 100 nM, non-essential amino acids solution 10 mM, Glutamax-I Supplement and Antibiotic-Antimycotic solution (all Thermo Fisher, Loughborough, UK). The media was supplemented with B-27 Supplement Minus Vitamin A, (Thermo Fisher), 20 ng/mL Human-EGF, 20 ng/mL Human-FGF-basic-154, 20 ng/mL Human-PDGF-AA, 20 ng/mL Human-PDGF-BB (all Shenandoah Biotech) and 2 µg/mL Heparin Solution (0.2%, Stem Cell Technologies). Cell authenticity was verified using short tandem repeat (STR) DNA fingerprinting. Cells were plated at a density of 1000–5000 cells/well on 96-well plates in a minimum of triplicates. After three days of incubation, the compound was added to each well in concentrations from 0.04–20000 nM and incubated at 37 °C, in 5% CO 2 , 95% humidity for eight days (192 h). For both sets of cell lines, cell viability was assessed by the 3D CellTiterGlo luminescent cell viability assay (Promega, G7573) and IC 50 values were calculated using GraphPad Prism version 8 as the concentration of compound required to reduce cell viability by 50%. Non-linear dose-response analysis with a four-parameter analysis (Inhibitor vs. Response–Variable Slope) was conducted using GraphPad Prism version 8 to fit a curve to the data. These IC 50 values for each cell line were then placed into one of two groups, wild-type or mutant, depending on PPM1D status. A parametric two-tailed t-test was run in Graphpad Prism version 8 to establish whether PPM1D -WT cell lines and PPM1D -mutant cell lines had significantly different IC 50 values. PPM1D and MDM2 cancer cell line dependency analysis The probability of dependency (PD) for all cell lines in the 18Q4 public release of the CRISPR-Avana pooled dependency screening database and associated mutation and copy number datasets were downloaded [17] , [18] . 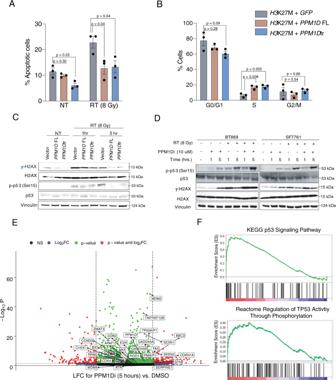Fig. 4:PPM1Dsuppresses apoptosis, DDR, and p53 pathways. Apoptosis and cell cycle responses were assessed in isogenic mouse neural stem cells (mNSCs) overexpressingH3F3AK27M (H3K27M) mutation plus either eGFP (vector control), full-lengthPPM1D(PPM1DFL), or C-terminus truncatedPPM1D(PPM1Dtr) (A–B).ACells were treated with 8 Gy of ionizing radiation (RT) or no treatment (NT) for 24 h, incubated with Annexin V-APC and Propidium Iodide (PI), and analyzed using flow cytometry. The total percentage of Annexin V positive cells representing both early and late apoptotic cells are shown. Data presented as mean ± SEM from three biological replicates.P= 0.027, 0.318, 0.044, 0.037 forGFPvsPPM1Dtr (NT),GFPvsPPM1DFL (NT),GFPvsPPM1Dtr (RT) andGFPvsPPM1D-FL (RT) conditions respectively calculated using two-tailed t-test.BCells were treated with 8 Gy RT for 24 h and integration of BrdU was assessed to determine the percentage of cells in S-phase. Anti-BrdU APC and 7-AAD DNA staining were used to distinguish cells in each stage of the cell cycle. Data presented as mean ± SEM from three biological replicates.P= 0.276, 0.090 0.008, 0.005, 0.543, 0.848 forGFPvsPPM1DFL (G0/G1)GFPvsPPM1Dtr (G0/1),GFPvsPPM1DFL (S)GFPvsPPM1Dtr (S),GFPvsPPM1DFL (G2/M)GFPvsPPM1Dtr (G2/M) conditions respectively calculated using two-tailedt-test.CCells were treated with 8 Gy of RT and lysates were collected at baseline (NT), 1 and 5 h post-RT respectively, and probed with the indicated antibodies. Three independent experiments were performed with similar results.DPPM1D-mutant patient-derived DMG cell lines BT869 and SF7761 were treated with 10 μM of GSK2830371 (PPM1Di) and/or 8 Gy of RT for 1 and 5 h, lysed and probed with indicated antibodies. Three independent experiments were performed with similar results.EVolcano plot showing differentially expressed genes in BT869 and SF7761 DMG cells (n= 3 per cell line per condition) treated with 10 μM of GSK2830371 (PPM1Di) for 5 h compared to vehicle treatment. Genes in the p53 signaling pathway are labeled.FGSEA enrichment plots of two p53 related pathways significantly enriched (FDR < 0.25) after inhibition of PPM1D in BT869 and SF7761 cells. Source data are provided as a Source Data file. PD for PPM1D was displayed for cell lines based on PPM1D mutational status, PPM1D copy-number, and TP53 mutational status. For pairwise gene-dependency, and MDM2 and PPM1D dependency correlation analyses, CERES scores from the 20Q1 public release of the DepMap dataset were used [17] . 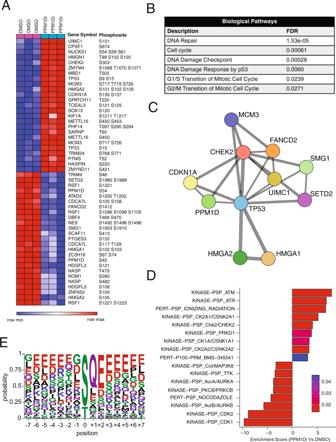Fig. 5: Phosphoproteomic analysis of PPM1D substrates inPPM1D-mutant cell lines. APatient-derivedPPM1D-mutant DMG cell line BT869 was treated with 10 μM of the PPM1D inhibitor GSK2830371 (or DMSO vehicle control) for 5 hours to suppress the PPM1D phosphatase following which phosphoproteomic profiling was performed.AHeatmap of top 50 differentially altered phosphosites (LFC > 1 and FDR < 0.01) between GSK2830371 treated (PPM1Di) and vehicle-treated (DMSO) samples is shown. Experiments were performed in triplicates.BPathway enrichment analysis using STRING reveals significantly associated biological pathways among phosphosites shown in (A) and, (C) Associated core interactome following PPM1D suppression.DSignificantly enriched or downregulated pathways (FDR < 0.05) revealed by PTM-SEA analysis of the phosphosites between the two conditions. Positive and negative enrichment scores correspond to biological pathways upregulated and downregulated respectively in GSK2830371 treated (PPM1Di) samples compared to vehicle-treated (DMSO) samples.EMotif analysis showing conserved amino acids flanking 97 confidently localized phosphorylation sites that are upregulated upon PPM1D inhibition in BT869 cells (LFC > 1, FDR < 0.01) and their associated probability of occurrence at that position. For PPM1D expression level, 20Q2 release of the expression dataset was used [18] . AUC for Nutlin-3 was obtained from PRISM Repurposing Secondary Screen 20Q2 release dataset [72] . Figures were made in R and GraphPad Prism. Quantification and statistical analysis Graphs showing quantification of Ki67 IHC staining were calculated from at least six individual tumors per condition, with 10 randomly selected fields imaged per sample. Cell viability curves for the different inhibitors were calculated from at least three independent experiments with triplicates for each condition. 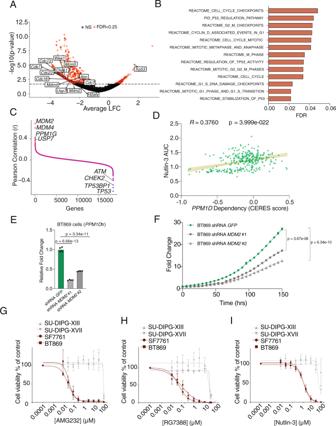Fig. 6: MDM2 inhibition is a dependency inPPM1D-mutant DMGs. AVolcano plot of genetic dependencies associated with mNSC overexpressingPPM1Dtr as revealed by genome-wide loss of function CRISPR-cas9 screen. Average LFC of normalized reads for each gene across three replicate experiments, and associated p-values are shown. A negative LFC represents depletion of guides across the assay. Genes that reach the FDR cutoff of 0.25 are labeled in red.BGene-sets significantly enriched (FDR < 0.05) within the dependencies associated withPPM1Dtr-expressing mNSCs following removal of pan-essential genes.CGenes ranked by Pearson correlation ofPPM1Ddependency (CERES score) against dependency of all other genes (CERES score) across 738 cancer cell lines.DCorrelation betweenPPM1Ddependency (CERES score) and response to Nutlin-3 treatment (AUC) across 309 cancer cell lines. Pearson correlation coefficient and associated two-tailed p-value of the coefficient are shown. Error bars represent 95% confidence interval.ERT-qPCR quantification ofMDM2expression in BT869 cell line infected with shRNA targeting GFP or MDM2 (two independent shRNA). Results show mean ± SEM for four replicates and are representative of three independent experiments.P= 6.66e−13 and 3.34e−11 forGFPvs shRNAMDM2#1 andGFPvs shRNAMDM2#2 respectively using two-tailedt-test.FGrowth of BT869 cells withMDM2knockdown from (E). Growth curves are mean ± SEM for at least three replicates and are representative of three independent experiments.P= 3.67e−08 and 6.34e−10 forGFPvs shRNAMDM2#1 andGFPvs shRNAMDM2#2 at 156 h respectively using two-tailedt-test.G–IDrug response curves for a panel of twoPPM1D-mutant and twoPPM1D-WT DMG cell lines treated with different concentrations ofMDM2inhibitors AMG232 (G), RG7388 (H), and Nutlin-3 (I) as indicated. Data presented as mean ± SEM from three independent experiments. Source data are provided as a Source Data file. 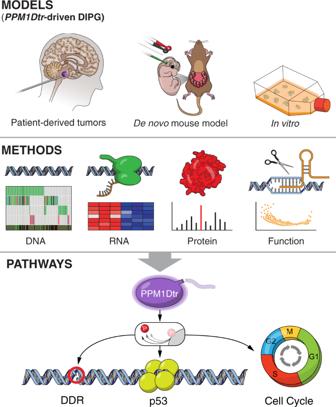Fig. 7: Integrative analysis ofPPM1D-mutant DMG models. Schematic depicting the overall method and findings of the study. Top panel: an array of models used in the study including biopsy of DMG tumors, de novo mouse models ofPPM1Ddriven DMG using in utero electroporation, and in vitro models including patient-derived cell lines. Middle panel: integrative approach employing whole-genome sequencing of patient tumors, gene expression analysis, proteomics, and phosphoproteomics screens, and CRISPR screens used to study the function and mechanism ofPPM1Dmutation in DMG. Bottom panel: convergence of the oncogenic function of PPM1Dtr on p53, cell cycle and DDR pathways using the integrative approach in the middle panel. Statistical significance was determined by Fisher’s exact test, Student’s t tests, log rank Mantel–Cox test, Kruskal–Wallis test, or Mann-Whitney test as indicated in the figure legends using Microsoft Excel, Graphpad Prism or R. Reporting summary Further information on research design is available in the Nature Research Reporting Summary linked to this article.